A lactate and formate transporter in the intraerythrocytic malaria parasite,Plasmodium falciparum The intraerythrocytic malaria parasite relies primarily on glycolysis to fuel its rapid growth and reproduction. The major byproduct of this metabolism, lactic acid, is extruded into the external medium. In this study, we show that the human malaria parasite Plasmodium falciparum expresses at its surface a member of the microbial formate–nitrite transporter family (PfFNT), which, when expressed in Xenopus laevis oocytes, transports both formate and lactate. The transport characteristics of PfFNT in oocytes (pH-dependence, inhibitor-sensitivity and kinetics) are similar to those of the transport of lactate and formate across the plasma membrane of mature asexual-stage P. falciparum trophozoites, consistent with PfFNT playing a major role in the efflux of lactate and hence in the energy metabolism of the intraerythrocytic parasite. The asexual intraerythrocytic form of the human malaria parasite Plasmodium falciparum relies primarily on glycolysis to meet its energy requirements [1] . Glucose is consumed by P. falciparum -infected erythrocytes at a rate some two orders of magnitude higher than by uninfected erythrocytes [2] . It enters the parasitized erythrocyte via a combination of the host cell’s endogenous glucose transporter and the parasite-induced ‘New Permeability Pathways’ [3] , and is then taken up into the parasite via the parasite’s plasma membrane hexose transporter [4] , [5] , [6] . Within the parasite, glucose is metabolized via glycolysis to lactic acid, which is excreted in large quantities from the parasite [2] via a H + -coupled transporter [7] , [8] , [9] . The P. falciparum genome contains genes for a number of candidate monocarboxylate transporters [10] , one of which is encoded by the gene PF3D7_0316600 (formerly PFC0725c). This protein falls within the microbial formate–nitrite family of transporters (FNT; TC 1.A.16), at least one other member of which has been shown to transport lactate and other products of anaerobic fermentation [11] , [12] . The protein encoded by PF3D7_0316600, referred to here as PfFNT ( P. falciparum Formate–Nitrite Transporter), was, together with P. falciparum hexose transporter and the nucleoside/nucleobase transporter PfENT1, one of the very few (putative or proven) transporter proteins detected in a proteomic analysis of a detergent-resistant membrane fraction prepared from mature blood-stage P. falciparum parasites [13] . This is perhaps indicative of it playing an important housekeeping role in the intraerythrocytic phase of the malaria parasite’s life cycle. In this study, we have explored the function and subcellular localization of this protein, and here present data implicating it in the transport of lactic acid and other monocarboxylic acids across the plasma membrane of the intraerythrocytic parasite. PfFNT has homologues in other apicomplexan parasites Formate/nitrite transporter homologues are present in a broad range of microbes but have not been identified in the animal or land plant genomes sequenced to date ( Supplementary Fig. 1 ). With the exception of Cryptosporidium species, all sequenced apicomplexan parasites harbour at least one FNT homologue, with the coccidian parasites (for example, Toxoplasma and Eimeria species) each encoding two or three FNT proteins and the haemosporidians and piroplasms (for example, Plasmodium and Theileria species) harbouring a single FNT homologue ( Supplementary Fig. 2 ). FNT homologues were not detected in the sequenced genomes of diplomonads ( Giardia ) or kinetoplastids ( Leishmania and Trypansoma ). The apicomplexan FNT homologues formed a monophyletic clade ( Supplementary Fig. 2 ), the topology of which is similar to current estimations of apicomplexan evolution [14] , [15] . This suggests that the FNT homologue was present early in the evolution of apicomplexans. Alignment of the sequence of PfFNT with a selection of homologues from other microorganisms revealed a number of conserved features ( Supplementary Fig. 3 ). For example, residues that have been implicated in the gating of the E. coli FocA transporter (T91, K156, E208, H209 and N213; ref. 16 ) are conserved in PfFNT. PfFNT transports formate and lactate The functional characteristics of PfFNT were investigated using the X. laevis oocyte expression system. cRNA encoding a carboxy terminal (C-terminal) hemagglutinin (HA)-tagged form of PfFNT (HA-PfFNT) was injected into X. laevis oocytes. Western blot analysis of an oocyte membrane preparation showed a band corresponding to ~32 kDa ( Fig. 1a ), very close to the predicted size of PfFNT (34 kDa). Immunofluorescence assay of oocytes expressing the tagged protein ( Fig. 1b ) revealed a fluorescent band external to the oocyte’s internal pigment layer, indicating that the protein is present in the oocyte plasma membrane. 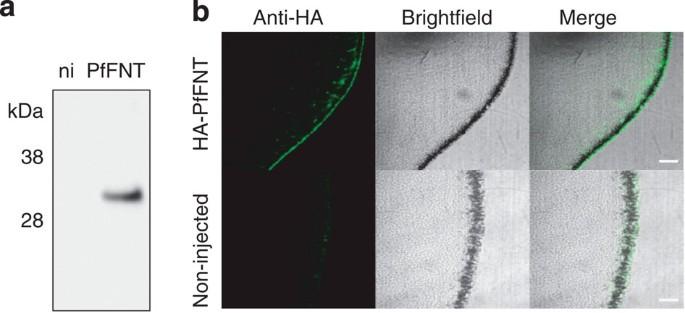Figure 1: Expression and localization of PfFNT inXenopus laevisoocytes. (a) Western blots of membranes from oocytes expressing C-terminal tagged HA-PfFNT, probed with an anti-HA antibody, show a band close to the predicted size of 34 kDa. The band is absent from membranes from non-injected (ni) oocytes. (b) Immunofluorescence images of oocytes injected with cRNA encoding C-terminal tagged HA-PfFNT show a clear band of fluorescence (corresponding to the plasma membrane) outside the pigment layer. The band is not seen in non-injected oocytes. Scale bar, 100 μm. In radiolabel uptake experiments, oocytes expressing the HA-tagged form of PfFNT accumulated [3H]formate to levels above those measured in non-injected oocytes, consistent with the tagged protein being functional. Figure 1: Expression and localization of PfFNT in Xenopus laevis oocytes. ( a ) Western blots of membranes from oocytes expressing C-terminal tagged HA-PfFNT, probed with an anti-HA antibody, show a band close to the predicted size of 34 kDa. The band is absent from membranes from non-injected (ni) oocytes. ( b ) Immunofluorescence images of oocytes injected with cRNA encoding C-terminal tagged HA-PfFNT show a clear band of fluorescence (corresponding to the plasma membrane) outside the pigment layer. The band is not seen in non-injected oocytes. Scale bar, 100 μm. In radiolabel uptake experiments, oocytes expressing the HA-tagged form of PfFNT accumulated [ 3 H]formate to levels above those measured in non-injected oocytes, consistent with the tagged protein being functional. Full size image Xenopus oocytes injected with cRNA encoding PfFNT showed a significant increase in the rate of uptake of both formate ( Fig. 2a ) and lactate ( Fig. 2b ) relative to non-injected controls. 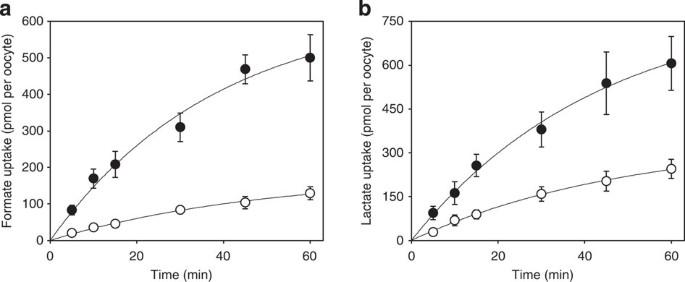Figure 2: Time courses for formate and lactate uptake inXenopusoocytes. Uptake of (a) formate and (b) lactate into PfFNT-expressing (closed circles) and non-injected (open circles) oocytes. Experiments were performed at 27.5 °C, pH 6.4, and an extracellular formate or lactate concentration of 1 mM. The data are averaged from those obtained in 4 independent experiments, each conducted on different days, using eggs from different frogs, and are shown ±s.e.m. Figure 2: Time courses for formate and lactate uptake in Xenopus oocytes. Uptake of ( a ) formate and ( b ) lactate into PfFNT-expressing (closed circles) and non-injected (open circles) oocytes. Experiments were performed at 27.5 °C, pH 6.4, and an extracellular formate or lactate concentration of 1 mM. The data are averaged from those obtained in 4 independent experiments, each conducted on different days, using eggs from different frogs, and are shown ±s.e.m. Full size image As is typically the case with the oocyte expression system (in which independent experiments are performed with oocytes from individual, unrelated frogs) there was substantial variability between experiments in the magnitude of the PfFNT-induced increase in the flux of formate and lactate. In oocytes expressing PfFNT, the rate of formate uptake was increased between 1.5- and 9.2-fold relative to the non-injected controls, with an average increase of 3.7±0.3-fold (mean±s.e.m. ; n =35; P <0.001, one-way analysis of variance (ANOVA)). The rate of lactate uptake was increased by between 1.1- and 4.4-fold relative to the non-injected controls, with an average increase of 3.1±0.3-fold ( n =13; P <0.001, one-way ANOVA). In paired experiments, the uptake of [ 14 C]formate into oocytes expressing PfFNT was comparable to that for oocytes expressing the rat monocarboxylate transporter rMCT1, whereas in oocytes expressing the unrelated P. falciparum (nucleoside/nucleobase) transporter PfENT1, formate uptake was similar to that in non-injected controls ( Supplementary Fig. 4 ; P >0.05, one-way ANOVA). PfFNT-induced transport is pH-dependent and inhibitable For both formate and lactate, PfFNT-induced uptake (calculated by subtracting uptake measured in non-injected oocytes from that measured in oocytes expressing PfFNT; Supplementary Fig. 5 ) increased with decreasing pH ( Fig. 3a ), consistent with (though not proof of) the transport of the two monocarboxylates being coupled to that of H + . The PfFNT-induced uptake of [ 14 C]formate was significantly reduced in the presence of a 10 mM concentration of lactate ( Fig. 3b ), as well as by a range of other carboxylates—pyruvate, acetate and propionate—and by the tricarboxylate citrate and the monovalent nitrite ion (each at 10 mM; Supplementary Fig. 6 ). The uptake of [ 14 C]lactate was similarly reduced in the presence of a 10 mM concentration of formate ( Fig. 3b ). These data are consistent with formate and lactate competing with one another for the transporter. 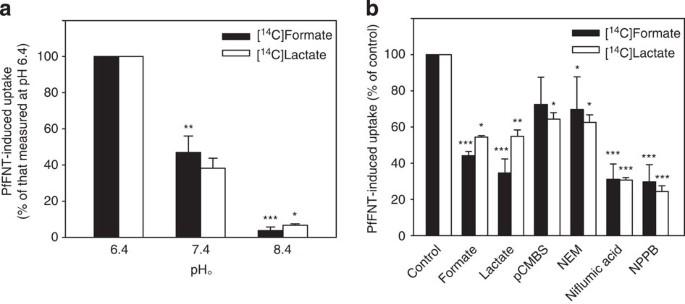Figure 3: Characteristics of formate and lactate uptake inXenopusoocytes. The (a) pH-dependence and (b) susceptibility to inhibition of PfFNT-induced formate and lactate uptake. Uptake was measured over 10 min at an extracellular formate or lactate concentration of 1 mM, except where specified otherwise. The data were averaged from those obtained innindependent experiments, each from different days, using eggs from different frogs, wherenwas: (a) 6 for [14C]formate (black bars) and 4 for [14C]lactate (white bars); (b) 4–8 for [14C]formate (black bars) and 4 for [14C]lactate (white bars). Inb, the extracellular pH was 6.4 and the potential competing substrates (formate and lactate; 10 mM) and inhibitors (100 μM) were added to the oocytes at the same time as the [14C]formate or [14C]lactate. In both panels, uptake is expressed relative to that measured at pH 6.4 in the absence of competing substrate or inhibitors. The asterisks denote statistical significance of the apparent differences between [14C]formate or [14C]lactate uptake measured under each of the different conditions tested and that measured in the relevant controls: *P<0.05; **P<0.01; ***P<0.001. Figure 3: Characteristics of formate and lactate uptake in Xenopus oocytes. The ( a ) pH-dependence and ( b ) susceptibility to inhibition of PfFNT-induced formate and lactate uptake. Uptake was measured over 10 min at an extracellular formate or lactate concentration of 1 mM, except where specified otherwise. The data were averaged from those obtained in n independent experiments, each from different days, using eggs from different frogs, where n was: ( a ) 6 for [ 14 C]formate (black bars) and 4 for [ 14 C]lactate (white bars); ( b ) 4–8 for [ 14 C]formate (black bars) and 4 for [ 14 C]lactate (white bars). In b , the extracellular pH was 6.4 and the potential competing substrates (formate and lactate; 10 mM) and inhibitors (100 μM) were added to the oocytes at the same time as the [ 14 C]formate or [ 14 C]lactate. In both panels, uptake is expressed relative to that measured at pH 6.4 in the absence of competing substrate or inhibitors. The asterisks denote statistical significance of the apparent differences between [ 14 C]formate or [ 14 C]lactate uptake measured under each of the different conditions tested and that measured in the relevant controls: * P <0.05; ** P <0.01; *** P <0.001. Full size image A range of pharmacological agents were tested for their effect on PfFNT-induced formate and lactate uptake ( Fig. 3b , with the effects on uptake into non-injected oocytes, and oocytes expressing PfFNT shown in Supplementary Fig. 7 ). The organo-mercurial reagent pCMBS (100 μM), an inhibitor of monocarboxylate transport in some cell-types [17] , and the sulfhydryl reagent N -ethylmaleimide (100 μM), both caused a modest inhibition of the PfFNT-induced uptake of formate and lactate. By contrast, the broad-specificity anion transport inhibitors niflumic acid (100 μM) and 5-nitro-2-(3-phenylpropylamino)benzoic acid (NPPB; 100 μM) caused a marked (~70%; P <0.05, one-way ANOVA) reduction in the PfFNT-induced uptake of the two monocarboxylates, while having a much lesser effect on the uptake of [ 14 C]formate into non-injected oocytes ( Supplementary Fig. 7 ). PfFNT-induced transport is saturable The concentration dependence of the PfFNT-induced uptake of formate and lactate uptake is shown in Fig. 4 , with the concentration dependence of uptake into non-injected oocytes and oocytes expressing PfFNT shown separately in the insets. The uptake of formate into non-injected oocytes ( Fig. 4a , inset) was a low-affinity process; a least-squares fit of the Michaelis–Menten equation to the data obtained over a formate concentration range of 0–10 mM yielded an ‘apparent K m ’ (25±5 mM) well above the maximum concentration tested. By contrast, PfFNT-induced formate uptake ( Fig. 4a ) showed a much higher affinity, with an estimated K m of 5.1±0.9 mM, and a mean V max of 528±83 pmol per oocyte per 10 min ( n =8). 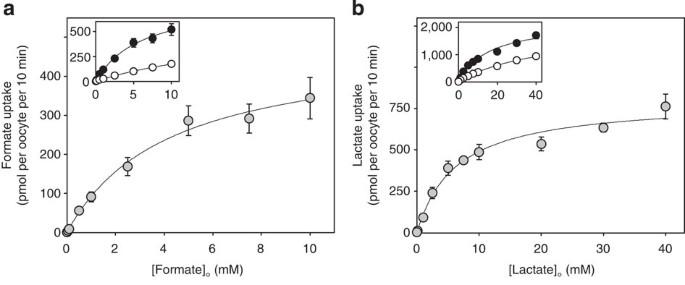Figure 4: Concentration dependence of PfFNT-induced formate and lactate uptake inXenopusoocytes. The PfFNT-induced uptake of formate (a) and lactate (b) was calculated by subtracting the uptake measured in non-injected oocytes (inset: open symbols) from that measured in oocytes expressing PfFNT (inset: closed symbols). The formate data are averaged from 8 independent experiments and the lactate data from 5 independent experiments, with each experiment done on a different day, using oocytes from different frogs, and shown ±s.e.m. The fitted curves were drawn using the Michaelis–Menten equation. Figure 4: Concentration dependence of PfFNT-induced formate and lactate uptake in Xenopus oocytes. The PfFNT-induced uptake of formate ( a ) and lactate ( b ) was calculated by subtracting the uptake measured in non-injected oocytes (inset: open symbols) from that measured in oocytes expressing PfFNT (inset: closed symbols). The formate data are averaged from 8 independent experiments and the lactate data from 5 independent experiments, with each experiment done on a different day, using oocytes from different frogs, and shown ±s.e.m. The fitted curves were drawn using the Michaelis–Menten equation. Full size image Similarly, the uptake of lactate into non-injected oocytes was a low-affinity process ( Fig. 4b inset), with an apparent K m (42±10 mM) well outside the concentration range tested. By contrast, PfFNT-induced lactate uptake ( Fig. 4b ) had an estimated K m of 7.3±1.7 mM and a V max of 834±83 pmol per oocyte per 10 min ( n =5). PfFNT is at the surface of the intraerythrocytic parasite The localization of PfFNT in asexual-blood-stage P. falciparum parasites was investigated by transfecting parasites with plasmids giving rise to the expression of either amino terminal (N-terminal) or C-terminal tagged HA-PfFNT. Western blots of membrane preparations from the transfected parasites revealed a band corresponding to 34 kDa ( Fig. 5a ), the predicted size of PfFNT. Immunofluorescence assay (using anti-HA antibodies) of erythrocytes infected with the transfectant parasites revealed fluorescence both in the vicinity of the parasite surface, consistent with a plasma membrane localization, and in the region surrounding the hemozoin crystals, consistent with the presence of the protein on the membrane of the parasite’s digestive vacuole (a lysosomal-type compartment; Fig. 5b ). The parasite surface localization of the protein was confirmed by co-localizing HA-PfFNT with the plasma membrane transporter PfENT1 (ref. 18 ; Fig. 5c ). Multiple attempts to confirm the localization by introducing an epitope tag through targeting the endogenous PfFNT locus proved unsuccessful. 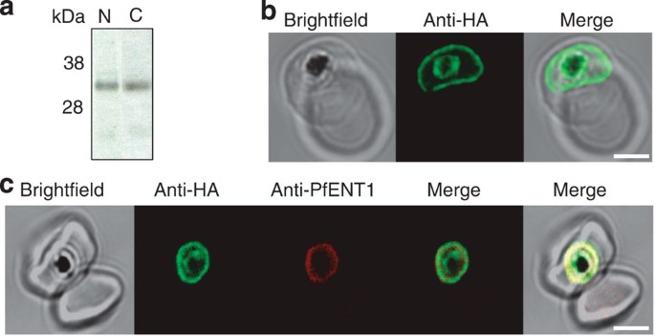Figure 5: Localization of HA-PfFNT in 3D7P. falciparumtrophozoites. (a) Western blot analysis of membrane preparations fromP. falciparumtrophozoites expressing either N-terminal or C-terminal tagged HA-PfFNT (lanes N and C, respectively), with a protein corresponding to the predicted size of 34 kDa identified in both cases. (b) An image of parasitized erythrocytes expressing C-terminal HA-tagged PfFNT, showing immunofluorescence both at the surface of the intraerythrocytic parasite and in the region surrounding the hemozoin crystals. Similar results were obtained with N-terminal HA-tagged PfFNT (not shown). (c) Co-localization of C-terminal tagged HA-PfFNT with the parasite’s plasma membrane nucleoside/nucleobase transporter PfENT1. Scale bar, 5 μm. Figure 5: Localization of HA-PfFNT in 3D7 P. falciparum trophozoites. ( a ) Western blot analysis of membrane preparations from P. falciparum trophozoites expressing either N-terminal or C-terminal tagged HA-PfFNT (lanes N and C, respectively), with a protein corresponding to the predicted size of 34 kDa identified in both cases. ( b ) An image of parasitized erythrocytes expressing C-terminal HA-tagged PfFNT, showing immunofluorescence both at the surface of the intraerythrocytic parasite and in the region surrounding the hemozoin crystals. Similar results were obtained with N-terminal HA-tagged PfFNT (not shown). ( c ) Co-localization of C-terminal tagged HA-PfFNT with the parasite’s plasma membrane nucleoside/nucleobase transporter PfENT1. Scale bar, 5 μm. Full size image Parasite formate transport resembles that via PfFNT Although the transport of lactate across the plasma membrane of the intraerythrocytic malaria parasite has been demonstrated and characterized previously [8] , [9] , that of the smaller formate ion has not. Formate was found here to traverse the parasite plasma membrane rapidly; in parasites functionally isolated from their host erythrocytes by saponin-permeabilization of the erythrocyte membrane and suspended at 4 °C and an extracellular pH of 6.1, [ 14 C]formate added to the extracellular medium reached a final distribution ratio (that is, the intracellular concentration relative to the extracellular concentration) of 2.7±0.1 (mean±s.e.m. ; n =4) within ~1 min ( Fig. 6a ). On raising the extracellular pH from 6.1 to 7.1, there was a marked decrease in the initial influx rate, as well as an ~10-fold decrease in the final distribution ratio ( Fig. 6b ). When the extracellular pH was increased further to 8.1, uptake of [ 14 C]formate was negligible ( Fig. 6b ). The pH-dependence of formate uptake into isolated parasites is consistent with formate uptake occurring via a H + -coupled mechanism. This was confirmed by the finding that addition of formate (10 mM) to isolated parasites, preloaded with the fluorescent pH-indicator BCECF, resulted in a rapid acidification ( Fig. 6c ), consistent with H + ions entering the parasite together with the formate. The uptake of formate into the isolated parasites was saturable, with a K m of 1.9 mM±0.7 and a V max of 9.2±1.8 pmol per 10 12 cells per hour ( Fig. 6d ). 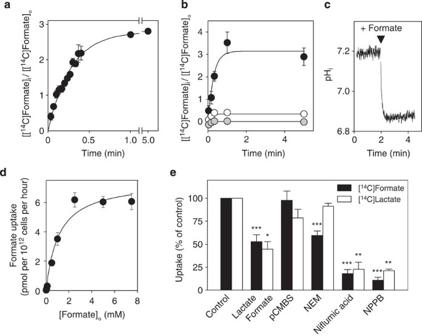Figure 6: Formate and lactate uptake into isolated 3D7P. falciparumtrophozoites. Unless specified otherwise, the extracellular pH was 6.1 and the extracellular formate concentration was 3.6 μM. (a) Time courses for [14C]formate uptake, shown as a ‘distribution ratio’ (that is, the intracellular concentration of radiolabel relative to that in the extracellular solution) and fitted to a first-order exponential equation. (b) pH-dependence of formate uptake. The parasites were suspended at an extracellular pH of 6.1 (black symbols), 7.1 (white symbols) or 8.1 (grey symbols) 10 min before the addition of [14C]formate. (c) Acidification of the cytosol of BCECF-loaded isolated parasites on addition of 10 mM formate to the extracellular medium (pH 7.1). (d) Concentration dependence of the uptake of formate (measured over 5 s), fitted to the Michaelis–Menten equation. (e) Effect of competing substrates (10 mM) and pharmacological agents (100 μM) on the uptake of formate (black bars) and lactate (external concentration 0.8 μM; white bars). The competing substrates and pharmacological agents were, in each case, added to the parasite suspension at the same time as the radiolabelled formate or lactate. Uptake was measured over either 5 or 20 s (both times fall within the initial, approximately linear phase of the uptake time course). Inc, data from a single representative experiment are shown. In the case of the other panels, the data were averaged from those obtained innindependent experiments, each from different days, wherenwas 4 ina; 3 inbfor the pH 6.1 and 7.1 data and 2 for the pH 8.1 data; 5 ind; 3–6 ine. The data are shown ±s.e.m (or, in the case of the pH 8.1 data inb, ±range/2). Ine, the asterisks denote the statistical significance of the apparent differences between [14C]formate or [14C]lactate uptake measured under each of the different conditions tested and that measured in the relevant ([14C]formate or [14C]lactate) control: *P<0.05; **P<0.01; ***P<0.001. Figure 6: Formate and lactate uptake into isolated 3D7 P. falciparum trophozoites. Unless specified otherwise, the extracellular pH was 6.1 and the extracellular formate concentration was 3.6 μM. ( a ) Time courses for [ 14 C]formate uptake, shown as a ‘distribution ratio’ (that is, the intracellular concentration of radiolabel relative to that in the extracellular solution) and fitted to a first-order exponential equation. ( b ) pH-dependence of formate uptake. The parasites were suspended at an extracellular pH of 6.1 (black symbols), 7.1 (white symbols) or 8.1 (grey symbols) 10 min before the addition of [ 14 C]formate. ( c ) Acidification of the cytosol of BCECF-loaded isolated parasites on addition of 10 mM formate to the extracellular medium (pH 7.1). ( d ) Concentration dependence of the uptake of formate (measured over 5 s), fitted to the Michaelis–Menten equation. ( e ) Effect of competing substrates (10 mM) and pharmacological agents (100 μM) on the uptake of formate (black bars) and lactate (external concentration 0.8 μM; white bars). The competing substrates and pharmacological agents were, in each case, added to the parasite suspension at the same time as the radiolabelled formate or lactate. Uptake was measured over either 5 or 20 s (both times fall within the initial, approximately linear phase of the uptake time course). In c , data from a single representative experiment are shown. In the case of the other panels, the data were averaged from those obtained in n independent experiments, each from different days, where n was 4 in a ; 3 in b for the pH 6.1 and 7.1 data and 2 for the pH 8.1 data; 5 in d ; 3–6 in e . The data are shown ±s.e.m (or, in the case of the pH 8.1 data in b , ±range/2). In e , the asterisks denote the statistical significance of the apparent differences between [ 14 C]formate or [ 14 C]lactate uptake measured under each of the different conditions tested and that measured in the relevant ([ 14 C]formate or [ 14 C]lactate) control: * P <0.05; ** P <0.01; *** P <0.001. Full size image The uptake of formate and lactate into isolated P. falciparum trophozoites was inhibited to a modest and somewhat variable extent by pCMBS (100 μM) and by N -ethylmaleimide (100 μM) and, as was seen for the PfFNT-induced uptake of both substrates into oocytes, to a much greater extent by niflumic acid (100 μM; P <0.01) and NPPB (100 μM; P <0.01, one-way ANOVA) ( Fig. 6e ). A comparison of the rates of uptake of formate and lactate into 3D7 parasites expressing N-terminal tagged HA-PfFNT with those into wild type 3D7 parasites revealed that, for both substrates, there was no significant difference between the two parasite lines ( Supplementary Fig. 8 ). Without a quantitative understanding of the relative levels of expression of the endogenous (untagged) FNT protein and the HA-tagged protein, or the relative transport activities of the untagged and tagged proteins, it is not possible to draw a definitive conclusion from these data. The characteristics of formate and lactate transport across the plasma membrane of isolated parasites are very similar to those of the PfFNT-induced transport of the two monocarboxylates in Xenopus oocytes. Both appear saturable with a K m in the low mM range; for formate the K m was 1.9 mM in the parasite (measured at 4 °C) and 5.1 mM in the oocyte (measured at 27.5 °C), while for lactate the K m (measured at 5 °C in a previous study [8] ) was 3.8 mM in the parasite and (as measured in this study at 27.5 °C) 7.3 mM in the oocyte. Both show similar pH-dependence, consistent with the transport being H + -coupled, and both were effectively inhibited by 100 μM concentrations of the anion transport blockers niflumic acid and NPPB. None of the inhibitors used in this study are specific; in particular, both niflumic acid and NPPB inhibit a range of anion transport pathways. Nevertheless, the fact that for both compounds the effect on formate/lactate transport in parasites is similar to that on PfFNT-induced transport in oocytes is at least consistent with PfFNT playing a role in the transport of monocarboxylates across the parasite plasma membrane. The marked similarities between the monocarboxylate transport characteristics observed in PfFNT-expressing Xenopus oocytes and in isolated parasites, together with the finding that PfFNT is localized to the parasite surface, are consistent with the hypothesis that PfFNT plays a major role in the flux of monocarboxylates across the parasite plasma membrane. From a physiological perspective, the primary monocarboxylate is lactate, excreted from the infected erythrocyte in large quantities as the end-product of the parasite’s anaerobic metabolism [2] . Formate is also present in significant quantities in asexual-stage P. falciparum parasites [19] . A recent study has highlighted the ability of a formate–nitrite transporter family member (FocA) from the enterobacterium Salmonella typhimurium to facilitate the export of the major end-products of anaerobic mixed-acid fermentation [11] . Such a role has not previously been demonstrated for eukaryote formate–nitrite transporter family members. However the findings here, consistent with PfFNT providing the major route for the transport of lactate across the plasma membrane of the intraerythrocytic (eukaryotic) malaria parasite, indicate that it may be more common than has previously been recognized. The formate–nitrite transporter family is unrelated to the monocarboxylate transporter family, members of which play the major role in the export of lactate from human cells. With the malaria parasite now showing resistance to most (if not all) antimalarials currently available, the revelation of such a fundamental biochemical difference between the parasite and its host, and the consequent potential of the PfFNT protein as an antimalarial drug target, is of obvious interest. A new paper by Beitz and colleagues reports the functional expression of PfFNT in yeast [20] . The authors present evidence that PfFNT transports lactate, formate and a number of other monocarboxylates via a coupled lactate:H + symport mechanism, and is localized to the parasite surface. The results of the study by Beitz and colleagues, obtained using a different expression system, are highly complementary to those presented here. Phylogenetic analysis of PfFNT FNT-family proteins were retrieved from the databases accessed at blast.ncbi.nlm.nih.gov/Blast.cgi , www.sanger.ac.uk/resources/downloads/protozoa/ , and www.eupathdb.org/eupathdb/ using a Basic Local Alignment Search Tool (BLAST) search and PfFNT as the query sequence. A representative selection of known and putative FNT homologues from a range of microorganisms were aligned using ClustalW [21] and the resulting alignments were manually adjusted in MacVector 12.7.5. Two proteins that are distantly related to the FNT family (from the flagellate protozoan Trichomonas vaginalis ; gi accession codes 123454345 and123479995) were included as an outgroup. Regions of the alignment that contained gaps or which could not be aligned unambiguously were excluded before analysis. Phylogenetic trees were estimated using the Neighbor-Joining method [22] and uncorrected amino acid distances in MacVector 12.7.5. Ties in the tree were resolved randomly and a bootstrap analysis [23] was performed with 1,000 pseudoreplicates. Cloning of PfFNT The gene encoding PfFNT was amplified from cDNA prepared from 3D7 parasites and inserted into the oocyte expression vector pGem-He-Juel [24] . The forward primer (5′-CC CCCGGG CCACC ATG CCACCAAATAATTCC)-3′ included an Ava I site (underlined) to enable further cloning as well as a short synthetic Kozak sequence (italicized) before the start codon (bold). The reverse primer (5′-G GAATTC TCA ATTTCGTAATTCTATAGAT)-3′ included an EcoR I site (underlined) and a stop codon (bold). C-terminally HA-tagged PfFNT was generated by PCR using the forward primer above and the reverse primer 5′-G GAATTC TTAAACAGCGTAATCTGGAACATCATATGGGTATGCAACAGC ATTTCTGAATTCTATAGAT-3′. The restriction enzyme site (underlined) was included and the HA-tag is shown in bold. All coding sequences were verified by sequencing. Expression of PfFNT and uptake of radiolabeled solutes in X. laevis oocytes In vitro transcription, oocyte preparation and cRNA injection (30 ng per oocyte) were performed as described elsewhere [25] . The mMessage mMachine T7 transcription kit and MEGAclear kit (Ambion) were used to produce cRNA. Oocytes were surgically removed from female X. laevis frogs and then collagen digested using collagenase D (Roche). Stage V & VI oocytes were manually selected for injection. The uptake into oocytes of [ 14 C]formate and [ 14 C]lactate was measured (4–6 days post injection) at 27.5 °C in media, which, unless specified otherwise, contained 96 mM NaCl, 2 mM KCl, 1 mM MgCl 2 , 1.8 mM CaCl 2 , 10 mM MES and 10 mM Tris-base, pH 6.4. Experiments were repeated using oocytes from different frogs (numbers are specified in the relevant figure legends), with each experiment using 8–10 oocytes for each condition tested. Western blotting and immunofluorescence in oocytes Membranes were isolated from twenty HA-tagged PfFNT-expressing oocytes as described elsewhere [25] . Briefly, 20 oocytes were homogenized in a homogenization buffer (10 mM NaCl, 1% Triton X-100 and 20 mM Tris-HCl), then centrifuged for 15 min, 15,000 g at 4 °C. A sample of the supernatant was diluted 1:12 then added to LDS NuPage buffer (Life Technologies) supplemented with 40 mM DTT and β-mercaptoethanol (1% v/v). Samples were separated on a 4–14% bis-Tris SDS/polyacrylamide gel (Life Technologies) and transferred onto nitrocellulose membranes. Western blots were carried out using a mouse anti-HA antibody (1:1,000) followed by horseradish peroxidase-conjugated goat anti-mouse antibody (1:10,000). Immunofluorescence analyses were performed on oocytes 5 days post injection using a protocol described elsewhere [25] . Mouse anti-HA antibodies (a gift from F. Shannon, Australian National University) (1:100), followed by Alexa Fluor 488 goat anti-mouse antibodies (Molecular Probes; 1:500) were applied to fixed oocytes. Oocytes were embedded in resin using the Technovit 7100 plastic embedding system (Kulzer) as described in detail elsewhere [26] and images of 4 μm slices were obtained on a Leica confocal microscope. For each condition, slices were viewed from at least three different oocytes, from at least two separate experiments using eggs from different frogs. Parasite culture P. falciparum parasites (3D7 strain [27] ) were maintained in continuous culture in Group O, Rh+ erythrocytes, as described previously [28] , with some modifications [29] , and were synchronized by sorbitol treatment [30] . Parasite transfection The MultiSite Gateway system (Life Technologies) was used to generate a transfection vector encoding a HA-tagged PfFNT protein. The coding sequence was amplified using the forward primer 5′- GGGGACACGTTTGTACAAAAAAGCAGGCT AAAATCCA ATG CCACCAAATAATTCC-3′, which contained the att1 site (underlined) and a start codon (bold). The reverse primer (5′- GGGGACCACTTTGTACAAGAAAGCTGGGT AACAGTATTTCGTAATTCTATAGAT-3′) contained the att2 site (underlined). The resulting sequence was inserted into the vector pDONR221 (Life Technologies) using a BP clonase reaction (Life Technologies). The Gateway LR clonase reaction (Life Technologies) was then used to recombine the PfFNT clone with a 5′ region from the gene encoding PfCRT ( P. falciparum chloroquine resistance transporter) and with a construct encoding a 3 × HA sequence. This generated a transfection vector that contained the gene encoding PfFNT, the PfCRT gene promoter and a sequence encoding the 3 × HA epitope tag (to be on either the N or C terminus of the recombinant protein). Constructs were transfected into 3D7 P. falciparum parasites using eletroporation, as described previously, with WR99210 (5 nM) used to select for transfectants [31] . Western blotting and immunofluorescence in parasites For immunofluorescence assays, fixed parasites were prepared using 4% w/v formaldehyde and 0.0075% w/v gluteraldehyde, as described elsewhere [31] . Fixed cells were blocked using 3% w/v BSA and mounted using SlowFade gold (Molecular Probes). Mouse anti-HA antibodies (a gift from F. Shannon, Australian National University) and rabbit PfENT1 antibodies (a gift from B. Ullman, Oregon Health and Science University) were used at a concentration of 1:200, followed by Alexa Fluor 488 goat anti-mouse antibodies (Molecular Probes) and Alexa Fluor 633 goat anti-rabbit antibodies (Life Technologies), respectively, each at a concentration of 1:1,000. Parasites were viewed on a Leica confocal microscope. For western blot analysis, a 10 ml parasitized erythrocyte suspension (15% parasitemia; 2–3% hematocrit) was centrifuged (3,000 g , 5 min) and the pellet resuspended in 1 ml of phosphate-buffered saline (PBS) supplemented with Complete-mini EDTA-free protease inhibitor cocktail. Saponin was added (to a final concentration of 0.09% w/v) to lyse the red blood cells and the sample was centrifuged (15,800 g , 5 min). The pellet was washed twice with PBS supplemented with the protease inhibitor cocktail and then triturated 15 times through a 25G syringe. A 15 μl aliquot was combined with 147.5 μl of PBS supplemented with protease inhibitor cocktail, 25 μl of β-mercaptoethanol (giving a final concentration of 10% v/v) and 62.5 μl NuPage sample loading buffer (giving a final concentration of 25% v/v). Western blot analysis was performed as described for the preparations of oocyte membrane protein. [ 14 C]Formate and [ 14 C]lactate uptake into isolated parasites Mature trophozoite-stage parasites (3D7 strain, ~36–40 h post invasion) were isolated from the contents of their host erythrocytes by brief exposure of the parasitized cells to saponin (final concentration 0.05% w/v, yielding a 0.005% w/v concentration of the active agent sapogenin), as described elsewhere [32] , [33] , [34] . Saponin renders the erythrocyte and parasitophorous vacuole membranes permeable to macromolecules [35] but leaves the parasite plasma membrane intact and able to maintain transmembrane ion gradients [32] , [33] , [34] , as well as a substantial membrane potential [36] . Following saponin treatment, the isolated parasites were washed (>3 times) and resuspended in a HEPES-buffered saline (125 mM NaCl, 5 mM KCl, 1 mM MgCl 2 , 20 mM glucose and 25 mM HEPES, pH 7.1). The uptake of [ 14 C]formate (and, in one series of experiments, [ 14 C]lactate) into isolated P. falciparum trophozoites was measured as described previously for nucleosides [37] . Briefly, uptake of [ 14 C]formate (or [ 14 C]lactate) was initiated by the addition of a 200 μl volume of a suspension of isolated parasites to an equal volume of radiolabeled substrate solution (at twice the intended final concentration) layered over a 200 μl dibutyl phthalate/dioctyl phthalate (5:4, v/v) oil mix. The final cell concentration was 0.5–1 × 10 8 cells ml −1 . All such experiments were carried out at 4 °C (in a cold room) to slow the rate of uptake. Uptake was stopped at predetermined times by sedimenting the parasites below the oil using centrifugation (15,800 g , 2 min) in a rapid-acceleration microcentrifuge (Beckman Microfuge E). Time points <15 s were sampled to the beat of a digital metronome. Where inhibitors or other substrates were used, these were added to the radiolabeled substrate solution before adding to the parasite suspension. The cell pellets were lysed using 0.1% (v/v) Triton X-100 and deproteinized with 5% w/v trichloroacetic acid before measuring the radioactivity in each sample using a scintillation counter [37] . Estimates of the amount of radioactivity present in the extracellular fluid trapped around the cell pellet was obtained by performing a short time course of radiolabelled uptake and extrapolating the time course data back to ‘time-zero’ [37] . The radioactivity in the extracellular fluid was subtracted from the total radioactivity in the pellet to provide an estimate of the amount of radiolabel within the cells. The concentration of radiolabel inside the cells was calculated by dividing the amount of radiolabel within the cells by the intracellular water volume of the pellet, calculated from the cell count using the previously reported value of 28 fL for the cell water volume of parasites isolated by saponin permeabilization of the host cell [38] . Time courses are presented in terms of ‘distribution ratios’ (that is, the estimated intracellular [ 14 C]formate concentration relative to the extracellular [ 14 C]formate concentration). pH measurements on isolated parasites The cytosolic pH (pH i ) of saponin-isolated trophozoite-stage parasites was measured (in parasites maintained at ~10 °C) using the ratiometric pH-sensitive fluorescent dye BCECF (Molecular Probes, Life Technologies), as described previously [33] . Statistics All errors cited and shown in the figures are s.e.m. All P values were obtained from one-way ANOVAs, using the pre-normalized uptake data (not the ‘% of control’ data). In the case of experiments with parasites, the ANOVA was followed by a post hoc Tukey test. In experiments with Xenopus oocytes, there was considerable variation in formate/lactate uptake in oocytes from different frogs (that is, considerable variation between independent experiments). To prevent the inter-experimental variation from eroding the precision of the test, we nominated ‘experiment’ as a ‘blocking factor’ in our one-way ANOVAs. When the ANOVA resulted in a P value <0.05, post hoc comparisons were performed using the least significant difference test. How to cite this article: Marchetti, R. V. et al. A lactate and formate transporter in the intraerythrocytic malaria parasite, Plasmodium falciparum . Nat. Commun. 6:6721 doi: 10.1038/ncomms7721 (2015).